Targeting TopBP1 at a convergent point of multiple oncogenic pathways for cancer therapy The progression of many solid tumours is driven by deregulation of multiple common pathways, particularly Rb, PI(3)K/Akt and p53. Prior studies identified TopBP1 as a key mediator for the oncogenic gain-of-function activities of mutant p53 (mutp53) in cancer. In Akt-hyperactive cancer, TopBP1 forms oligomers and represses E2F1-dependent apoptosis. Here we perform a molecular docking screening and identify a lead compound, calcein, capable of blocking TopBP1 oligomerization and p53 binding, resulting in re-activation of E2F1-dependent apoptosis and blockade of mutp53 gain-of-function. Calcein AM, the cell-permeable derivative of calcein, shows significant antitumour activity in a wide spectrum of cultured cancer cells harbouring high TopBP1 levels. These biochemical findings are recapitulated in breast cancer xenograft models. Thus, our study provides proof-of-concept evidence for targeting TopBP1, a convergent point of multiple pathways, as a cancer therapy. Despite the complexity of mutations in different cancers, recent efforts in cancer genome sequencing project have shown that a handful of core signalling pathways, such as receptor tyrosine kinases (RTK)/RAS/phosphatidylinositol 3-kinase (PI(3)K), p53 and retinoblastoma (Rb) protein, are deregulated in majority of solid tumours. For example, 77% of breast cancers have genetic alterations in the PI(3)K/Akt pathway, and 49% have alterations in p53 signalling [1] . Particularly in basal-like breast cancer (often triple-negative breast cancer or TNBC), 84% show TP53 mutations, 35% show PTEN mutation/loss and 20% show RB1 mutation/loss [1] . These deregulated signalling pathways often converge to some common modulators. As a key regulator for cell growth, the Rb pathway is deregulated in most cancers, resulting in high E2F1 activities to drive cell cycle progression. E2F1 also has a pro-apoptotic role through activating target genes such as TP73 (ref. 2 , 3 ), Apaf-1 and caspases [4] , [5] during DNA damage [6] . How to activate E2F1 pro-apoptotic activity inside cancer cells remains an elusive goal. Previously, we showed that a checkpoint activator protein, topoisomerase IIβ-binding protein 1 (TopBP1), plays a critical role in suppressing E2F1 pro-apoptotic activity in response to PI(3)K/Akt signalling, which suggests TopBP1 as a therapeutic target to activate E2F1-dependent apoptosis in cancer [7] , [8] , [9] , [10] . TopBP1 utilizes its multiple BR CA1 c arboxyl- t erminal (BRCT) motifs as scaffolds to modulate many processes of DNA metabolism, such as DNA damage checkpoint, replication and transcription [11] . TopBP1 represses E2F1 transcriptional activities by recruiting the Brg1/Brm chromatin remodelling complex [8] . TopBP1 also binds the DNA-binding domain (DBD) of p53 to inhibit its transcriptional function [12] . Regulation of E2F1 and p53 by TopBP1 is important to control the pro-apoptotic activities of both transcription factors during normal S phase transition. While TopBP1 is involved in seemingly separate functions, our recent study showed that its functions in replication checkpoint and transcriptional regulation are indeed coordinated via an Akt-dependent conformational change of TopBP1 (ref. 10 ). Akt phosphorylates TopBP1 at Ser1159 and induces its oligomerization through an intermolecular interaction between the phosphorylated Ser1159 residue (pS1159) and the 7–8th BRCT (BRCT7/8) domain of two TopBP1 molecules [9] , [10] . Oligomerization of TopBP1 then induces its binding to E2F1, but at the same time prevents its recruitment to chromatin and ATR binding and perturbs its checkpoint-activating functions [10] . Thus, by regulating TopBP1 quaternary structure, Akt switches TopBP1 function from checkpoint activation to transcriptional regulation. This mechanism is responsible for inhibition of E2F1-dependent apoptosis (an oncogenic checkpoint) and inhibition of ATR function (replication checkpoint) in the tumours with high Akt activity. Therefore, selective blockade of TopBP1 oligomerization may provide a novel therapeutic strategy in cancer cells that exhibit upregulated PI3K/Akt signalling. Many mutant p53 proteins do not only lose normal p53 function but also gain new functions that contribute to cancer progression (‘gain-of-function’ activities (GOF)) [13] , [14] . In addition to mutations, cancer cells can have a different mechanism to inactivate p53: upregulation of p53-negative regulators, such as MDM2 (ref. 15 ), MDMX [16] and TopBP1 (ref. 12 ). Adding to the complexity of p53 regulation is the presence of 12 p53 isoforms with differential expression [17] , some of which have dominant-negative activities against p53 (ref. 18 ). TopBP1 also mediates mutp53 GOF by facilitating its complex formation with NF-Y and p63/p73 (ref. 19 ). Since TopBP1 is an E2F target [8] , it is often upregulated upon inactivation of the Rb pathway [12] . Indeed, TopBP1 is frequently overexpressed in breast cancer and its overexpression is associated with a shorter survival [12] , [19] . Single-nucleotide polymorphisms (SNPs) in TopBP1 that cause higher expression of TopBP1 mRNA and protein have also been associated with an increased risk in breast and endometrial cancers [20] , [21] . Thus, deregulation of the Rb pathway may be functionally linked to mutp53 and be responsible for at least part of mutp53 GOF via TopBP1. The accumulated TopBP1 in cancer cells then inhibits growth checkpoints through repressing E2F1 and p53 functions, and collaborates with mutp53 to further promote tumour progression. Therefore, TopBP1 might be a target among the nexus of these major oncogenic pathways. Here we perform a molecular docking screening and identify calcein as a compound to target the BRCT7/8 domain of TopBP1. We also use its cell-permeable derivative Calcein AM to provide proof-of-principle evidence for targeting TopBP1 as a cancer therapy. Calcein blocks oligomerization and p53 binding of TopBP1 On the basis of the mechanisms of action, we sought to design the TopBP1 inhibitors capable of blocking TopBP1 oligomerization and its interaction with mutp53. Since the BRCT7/8 domains of TopBP1 are responsible for both oligomerization and binding to p53 (ref. 12 ), and the BRCT domains form structured binding pockets, TopBP1-BRCT7/8 would be the ideal domains for screening compounds that block TopBP1 binding to pS1159 peptide and mutant p53. Using the TopBP1-BRCT7/8 structure [22] , we performed a molecular docking screening to identify compounds that can bind to TopBP1-BRCT7/8. From a library of more than 2,000 compounds including Food and Drug-approved drugs (Microsource Spectrum Collection), we identified 61 compounds with top scores for fitting into the structural pocket of TopBP1-BRCT7/8 and with molecular weights of greater than 250 g. We then performed biochemical binding assays (pS1159 peptide-binding assay [10] and glutathione S-transferase (GST)-p53(DBD) pulldown assay [12] ) to test the ability of these 61 compounds to block the interactions between TopBP1-BRCT7/8 and pS1159 peptide or p53(DBD). The compounds that showed activities in the initial screening were subjected to multiple independent binding assays for reproducibility. We identified an oxospiro-benzofuran derivative compound, calcein ( Fig. 1a ), that blocked the interactions of TopBP1-BRCT7/8 with pS1159 peptide ( Fig. 1b ) and p53(DBD) ( Fig. 1c ). The docking of calcein into the TopBP1-BRCT7/8 pocket viewed from two different angles is shown in Fig. 1d,e . As seen from Fig. 1e , calcein is predicted to form H-bonds with K1317, R1280, S1273, S1274, R1314 and R1407, among which K1317 and S1273 had been demonstrated to be important for binding to pS1159 for oligomerization [10] . We also tested these candidates in E2F1 activity reporter assay [7] and p53 activity reporter assay [12] . Calcein is a hydrophilic fluorescent molecule that does not get into cells. Its nonfluorescent acetomethoxy derivative, Calcein AM (acetoxymethyl ester), can enter cells where it is hydrolysed by esterases to calcein and retains inside the cells. We therefore used Calcein AM for cell culture experiments. Among these potential compounds, Calcein AM stood out in its ability to induce both E2F1 ( Supplementary Fig. 1 ) and p53 activities ( Supplementary Fig. 2 ). Both pS1159 peptide binding and GST-p53(DBD) pulldown assays showed that calcein blocked the TopBP1/pS1159 interaction ( Fig. 1f ) and TopBP1/p53(DBD) interaction ( Fig. 1g ) at submicromolar concentrations. 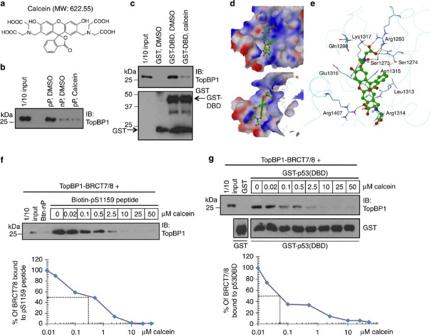Figure 1: Calcein binds TopBP1-BRCT7/8 and inhibits its binding to the pS1159 peptide and p53-DBD. (a) Structure of calcein, a fluorescent molecule with formula C30H26N2O13and molecular weight 622.55. (b) Purified TopBP1-BRCT7/8 was incubated with DMSO or calcein and Btn-pS1159 peptide phosphorylated peptide (pP) or nonphosphorylated peptide (nP), followed by streptavidin Sepharose pulldown as described in the Methods9. The pulldown TopBP1-BRCT7/8 was analysed by western blotting (IB) with a TopBP1 antibody (BL893, Bethyl Laboratories), which recognizes the C terminus of TopBP1. The result was replicated three times. (c) Purified TopBP1-BRCT7/8 was incubated GST-p53(DBD) in the presence of DMSO or calcein, and GST pulldown assay was performed12. This result was replicated four times. (d) The lowest-energy docking position of calcein (ball and stick model) in the structure of TopBP1-BRCT7/8 (shown as an electrostatic molecular surface), viewed from two different angles, shows favourable multiple polar and hydrophobic interactions between BRCT7/8 and calcein with a large aromatic system. (e) The interactions between the docked structure of calcein and the adjacent residues of TopBP1. H-bonds are shown as dotted lines. (f) Streptavidin Sepharose pulldown as inbwas performed in the presence of various concentrations of calcein. (g) GST-p53(DBD) pulldown assay as incwas performed in the presence of various concentrations of calcein. Figure 1: Calcein binds TopBP1-BRCT7/8 and inhibits its binding to the pS1159 peptide and p53-DBD. ( a ) Structure of calcein, a fluorescent molecule with formula C 30 H 26 N 2 O 13 and molecular weight 622.55. ( b ) Purified TopBP1-BRCT7/8 was incubated with DMSO or calcein and Btn-pS1159 peptide phosphorylated peptide (pP) or nonphosphorylated peptide (nP), followed by streptavidin Sepharose pulldown as described in the Methods [9] . The pulldown TopBP1-BRCT7/8 was analysed by western blotting (IB) with a TopBP1 antibody (BL893, Bethyl Laboratories), which recognizes the C terminus of TopBP1. The result was replicated three times. ( c ) Purified TopBP1-BRCT7/8 was incubated GST-p53(DBD) in the presence of DMSO or calcein, and GST pulldown assay was performed [12] . This result was replicated four times. ( d ) The lowest-energy docking position of calcein (ball and stick model) in the structure of TopBP1-BRCT7/8 (shown as an electrostatic molecular surface), viewed from two different angles, shows favourable multiple polar and hydrophobic interactions between BRCT7/8 and calcein with a large aromatic system. ( e ) The interactions between the docked structure of calcein and the adjacent residues of TopBP1. H-bonds are shown as dotted lines. ( f ) Streptavidin Sepharose pulldown as in b was performed in the presence of various concentrations of calcein. ( g ) GST-p53(DBD) pulldown assay as in c was performed in the presence of various concentrations of calcein. Full size image Ironically, Calcein AM was developed as a cell viability assay, since only live cells can hydrolyse nonfluorescent Calcein AM into fluorescent calcein and retain calcein inside the cells. Calcein AM treatment was reported to have cytotoxic effect in some cancer cells [23] , [24] , [25] ; nevertheless, its detailed mechanisms of action remain unclear. We used Calcein AM to further investigate the in vivo effect of calcein in TopBP1 signalling. Since the interaction between TopBP1-BRCT7/8 and pS1159 peptide mediates TopBP1 oligomerization [10] , Calcein AM was expected to block TopBP1 oligomerization. Indeed, using differentially tagged TopBP1, we found that Calcein AM (2.5 μM) was able to inhibit TopBP1 oligomerization in triple-negative, PTEN -null MDA-MB468 breast cancer cells ( Fig. 2a ). Calcein AM also blocked endogenous TopBP1 oligomerization in a dimethyl pimelimidate-2HCl (DMP) chemical crosslinking assay [10] ( Fig. 2b ). Here MK2206, an Akt allosteric inhibitor, was used as a positive control for blocking Akt-dependent TopBP1 oligomerization [10] . Importantly, Calcein AM not only inhibited the interaction between overexpressed E2F1 and TopBP1 in HEK293T cells ( Fig. 2c ) but also inhibited TopBP1/E2F1 and TopBP1/mutp53 interactions in MDA-MB468 cells (harbouring mutp53(R273H)) at physiological levels ( Fig. 2d ). TopBP1/mutp53 interaction has been shown to facilitate the binding of mutp53 to p63/p73 (ref. 19 ). Calcein AM treatment also led to the release of p73 from mutp53 ( Fig. 2e ). 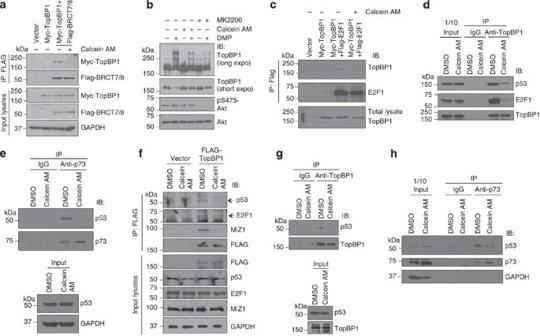Figure 2: Calcein inhibits TopBP1 oligomerization and binding to E2F1 and mutp53 and disrupts the interaction of mutp53 from p73. (a) MDA-MB468 cells were transfected with Myc-TopBP1 alone and in combination with FLAG-TopBP1-BRCT7/8. Cells were treated with Calcein AM (2.5 μM) or DMSO for 5 h. Cells were then lysed and immunoprecipitated with anti-FLAG beads followed by immunoblotting as described10. (b) MDA-MB468 cells were treated with Calcein AM (2.5 μM) or DMSO for 5 h and then lysed and incubated with 20 mM DMP for 30 min following the crosslinking protocol described in the Methods section. Cell lysates were analysed by SDS–PAGE and immunoblotted with indicated antibodies. MK2206 (1 μM for 24 h) served as a positive control10. The result was replicated for three times. (c) HEK293 cells expressing Myc-TopBP1 and FLAG-E2F1 were treated with Calcein AM or DMSO for 5 h, followed by immunoprecipitation and immunoblotting as indicated. (d) MDA-MB468 cells were treated with Calcein AM (2.5 μM) or DMSO for 5 h. The cell lysates were then subjected to immunoprecipitation with anti-TopBP1 antibody or control mouse IgG and then immunoblotting to detect interacting mutp53 and E2F1. This result was replicated for three times. (e) MDA-MB468 cells were treated with Calcein AM (2.5 μM) or DMSO for 5 h. The cell lysates were then subjected to immunoprecipitation with anti-p73 antibody or control mouse IgG and then to immunoblotting to detect mutp53. (f) BT549 cells were transfected with FLAG-TopBP1 or an empty vector. Two days later, cells were treated with Calcein AM (2.5 μM) or DMSO for 3 h and then harvested for anti-FLAG immunoprecipitation10. (g) The interaction of endogenous TopBP1 and mutp53 in BT549 cells was examined by co-immunoprecipitation using anti-TopBP1 antibody or a control mouse IgG after cells were treated with Calcein AM (2.5 μM) or DMSO for 5 h. (h) BT549 cells were treated with Calcein AM (2.5 μM) or DMSO for 5 h, and then subjected to anti-p73 (or a control mouse IgG) immunoprecipitation. Figure 2: Calcein inhibits TopBP1 oligomerization and binding to E2F1 and mutp53 and disrupts the interaction of mutp53 from p73. ( a ) MDA-MB468 cells were transfected with Myc-TopBP1 alone and in combination with FLAG-TopBP1-BRCT7/8. Cells were treated with Calcein AM (2.5 μM) or DMSO for 5 h. Cells were then lysed and immunoprecipitated with anti-FLAG beads followed by immunoblotting as described [10] . ( b ) MDA-MB468 cells were treated with Calcein AM (2.5 μM) or DMSO for 5 h and then lysed and incubated with 20 mM DMP for 30 min following the crosslinking protocol described in the Methods section. Cell lysates were analysed by SDS–PAGE and immunoblotted with indicated antibodies. MK2206 (1 μM for 24 h) served as a positive control [10] . The result was replicated for three times. ( c ) HEK293 cells expressing Myc-TopBP1 and FLAG-E2F1 were treated with Calcein AM or DMSO for 5 h, followed by immunoprecipitation and immunoblotting as indicated. ( d ) MDA-MB468 cells were treated with Calcein AM (2.5 μM) or DMSO for 5 h. The cell lysates were then subjected to immunoprecipitation with anti-TopBP1 antibody or control mouse IgG and then immunoblotting to detect interacting mutp53 and E2F1. This result was replicated for three times. ( e ) MDA-MB468 cells were treated with Calcein AM (2.5 μM) or DMSO for 5 h. The cell lysates were then subjected to immunoprecipitation with anti-p73 antibody or control mouse IgG and then to immunoblotting to detect mutp53. ( f ) BT549 cells were transfected with FLAG-TopBP1 or an empty vector. Two days later, cells were treated with Calcein AM (2.5 μM) or DMSO for 3 h and then harvested for anti-FLAG immunoprecipitation [10] . ( g ) The interaction of endogenous TopBP1 and mutp53 in BT549 cells was examined by co-immunoprecipitation using anti-TopBP1 antibody or a control mouse IgG after cells were treated with Calcein AM (2.5 μM) or DMSO for 5 h. ( h ) BT549 cells were treated with Calcein AM (2.5 μM) or DMSO for 5 h, and then subjected to anti-p73 (or a control mouse IgG) immunoprecipitation. Full size image Previously, we showed that TopBP1 can interact with both ‘contact mutant’ p53 (such as R273H) and conformational mutants (such as R175H and R249S) [19] . Thus, we also tested Calcein AM in another triple-negative, PTEN -null breast cancer cell line BT549, which contains a conformational mutant R249S mutp53. Calcein AM treatment inhibited the interaction between TopBP1 and mutp53 and E2F1 in BT549 cells ( Fig. 2f,g ). Consistent with a role for TopBP1 oligomerization [9] , Calcein AM also inhibited the interaction between TopBP1 and Miz1 ( Fig. 2f ), suggesting that the release of Miz1 from TopBP1 might mediate some of Calcein AM activities. Importantly, Calcein AM treatment also resulted in the release of p73 from mutp53(R249S) in BT549 cells ( Fig. 2h ) like it did in MDA-MB468 cells. Calcein AM activates E2F1 and p53 and blocks mutp53 GOF Next, we examined the effect of Calcein AM on E2F1 and p53 transcriptional activities using E2F1 (ref. 7 ) and p53 activity reporter assay [12] , respectively. In line with its effect on blocking TopBP1 function in repressing E2F1 and p53 activities, Calcein AM treatment enhanced E2F1 and p53 transcriptional activities ( Fig. 3a,b ). To demonstrate that the induction of p14 Arf promoter-luciferase activity by Calcein AM was indeed because of E2F1, we performed an independent assay using a pair of the p68 subunit of DNA polymerase α promoter constructs: pKL12 (containing two wild-type E2F sites) and pKL12-E2FAB (both E2F sites being mutated and no longer responding to E2F) [7] , [26] . Indeed, Calcein AM could only induce the activity on pKL12, but not on pKL12-E2FAB ( Supplementary Fig. 3 ). To show that the induction of p21 promoter activity by Calcein AM was dependent on p53, we used a pair of isogenic cell lines [27] p53 +/+ and p53 −/− HCT116 and showed that the induction of p21 and another p53 target Bax was observed on in p53 +/+ , but not in p53 −/− HCT116 cells ( Supplementary Fig. 4 ). Previously using a p73 activity reporter (Bax-promoter-driven luciferase) assay, we found that in p53-null H1299 cells, overexpression of mutp53(R273H) blocked the p73 transcriptional activity in a TopBP1-dependent manner [19] . Consistently, mutp53(R273H) inhibited p73 transcriptional activity, and indeed this activity was blocked by Calcein AM ( Fig. 3c ), indicating an inhibitory effect of Calcein AM on mutp53 GOF. To further investigate whether Calcein AM affected endogenous activities of E2F1 and mutant p53, we examined the target genes of E2F1, p63/p73 and NF-Y in MDA-MB468 cells. Calcein AM upregulated E2F1 pro-apoptotic target genes, such as TP73 , Apaf-1 and Caspase 3 in MDA-MB468 cells ( Fig. 3d ). Calcein AM also inhibited mutp53 GOF activities by the upregulation of p63/p73 target genes such as Bax , Noxa , Hdm2 and downregulation of NF-Y target genes, such as Cdk1 , Cdc25C and Cyclin A2 (ref. 19 ; Fig. 3d ). These data demonstrate that calcein binds TopBP1 to block mutp53 GOF and restore pro-apoptotic activities of E2F1 and p63/p73. 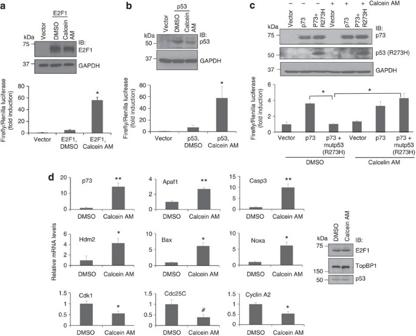Figure 3: Calcein AM induces E2F1 and p53 activities and blocks mutp53 gain-of-function. (a) E2F1 transcriptional activity was measured by a p14Arfpromoter dual luciferase assay in HEK293 cells7after Calcein AM treatment. The normalized activities of E2F1 were shown as fold induction relative to that of the empty vector control. Results shown are the means±s.d. from three independent experiments (biological replicates). *P<0.001 (two-tailedt-test). (b) p53 transcriptional activity was measured by a p21 promoter dual luciferase assay in H1299 cells12after Calcein AM treatment. The normalized activities of p53 (means±s.d. from three biological replicates) were shown as fold induction relative to that of the empty vector control. *P<0.05 (two-tailedt-test). (c) The effect of Calcein AM on mutp53(R273H) gain-of-function was measured in p53-null H1299 cells expressing p73α and mutp53 (R273H), along with a p73 activity reporter plasmid (a Bax promoter-luciferase plasmid) and pRL-TK as described19. Luciferase activity of transfected p73 was determined as fold induction relative to that of the empty vector control (means±s.d. from three biological replicates). A portion of the cell lysates was subjected to immunoblotting with the indicated antibody (upper panel). *P<0.001 (two-tailedt-test). (d) MDA-MB468 cells were treated with Calcein AM as inFig. 2d. RNA was then isolated for real-time RT–PCR analysis using primers specific to E2F1, p53 and NF-Y target genes or GAPDH. Results were normalized to GAPDH levels and the means±s.d. (n=3) are expressed relative to the expression of genes in control cells. Aliquots of the cell lysates were analysed by immunoblotting (right panel). The experiment was performed in biological triplicates.**P<0.001; *P<0.01;#P<0.05 (two-tailedt-test). Figure 3: Calcein AM induces E2F1 and p53 activities and blocks mutp53 gain-of-function. ( a ) E2F1 transcriptional activity was measured by a p14 Arf promoter dual luciferase assay in HEK293 cells [7] after Calcein AM treatment. The normalized activities of E2F1 were shown as fold induction relative to that of the empty vector control. Results shown are the means±s.d. from three independent experiments (biological replicates). * P <0.001 (two-tailed t -test). ( b ) p53 transcriptional activity was measured by a p21 promoter dual luciferase assay in H1299 cells [12] after Calcein AM treatment. The normalized activities of p53 (means±s.d. from three biological replicates) were shown as fold induction relative to that of the empty vector control. * P <0.05 (two-tailed t -test). ( c ) The effect of Calcein AM on mutp53(R273H) gain-of-function was measured in p53-null H1299 cells expressing p73α and mutp53 (R273H), along with a p73 activity reporter plasmid (a Bax promoter-luciferase plasmid) and pRL-TK as described [19] . Luciferase activity of transfected p73 was determined as fold induction relative to that of the empty vector control (means±s.d. from three biological replicates). A portion of the cell lysates was subjected to immunoblotting with the indicated antibody (upper panel). * P <0.001 (two-tailed t -test). ( d ) MDA-MB468 cells were treated with Calcein AM as in Fig. 2d . RNA was then isolated for real-time RT–PCR analysis using primers specific to E2F1, p53 and NF-Y target genes or GAPDH. Results were normalized to GAPDH levels and the means±s.d. ( n =3) are expressed relative to the expression of genes in control cells. Aliquots of the cell lysates were analysed by immunoblotting (right panel). The experiment was performed in biological triplicates. ** P <0.001; * P <0.01; # P <0.05 (two-tailed t -test). Full size image Calcein AM kills TopBP1-overexpressing cancer cells We then performed MTS assay to determine the cytotoxic activity of Calcein AM in three breast cancer cell lines MDA-MB468, MDA-MB231 and MCF7 and a nontransformed MCF10A cell line. Calcein AM preferentially inhibited the proliferation of these three cancer cell lines ( Fig. 4a ). The caspase 3/7 activity assay showed that Calcein AM-induced apoptosis in MCF7, MDA-MB231 and MDA-MB468 cells, but to a much lesser degree in MCF10A cells ( Fig. 4b ). When co-treated with doxorubicin (adriamycin), Calcein AM greatly enhanced the doxorubicin sensitivity in MDA-MB468, but not in MCF10A cells ( Fig. 4c and Supplementary Fig. 5 ). Mutp53 GOF has been shown to expand the breast cancer stem cells [28] , which form mammospheres in suspension culture [29] . The mammosphere formation of MDA-MB468 cells was also blocked by Calcein AM ( Fig. 4d ). It is possible that this is at least in part because of the cytotoxic activity of Calcein AM, but at the concentration used in this experiment, many cells still survived and could be scored ( Supplementary Fig. 6 ); however, they failed to form mammosphere. To further investigate the cytostatic (inhibiting proliferation) and cytotoxic (inducing apoptosis) activities of Calcein AM in a quantitative way, we performed colony formation assay ( Fig. 4e and Supplementary Fig. 7 ) and caspase 3/7 activity assay ( Fig. 4f ) after treating MDA-MB468 cells with increasing doses of Calcein AM. While apoptosis was induced at 2.5 and 5 μM, but not at 0.1 and 0.5 μM, inhibition of colony formation was apparent at 0.1 μM and beyond. Thus, Calcein AM exerts its effect through its activity in suppressing proliferation and, when given at higher doses, inducing apoptosis. 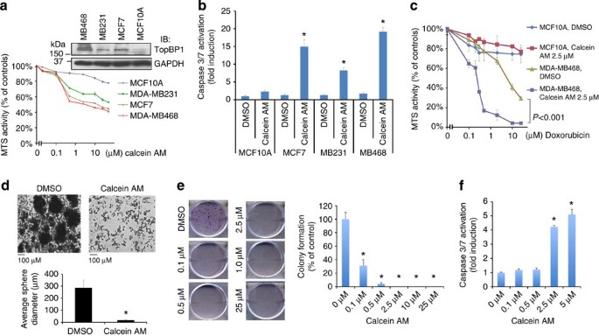Figure 4: Calcein AM shows antitumour activity against many different cancer cell lines. (a) MTS assays were performed in breast cancer cell lines MDA-MB468, MDA-MB231 and MCF7, and nontransformed breast epithelial cell line MCF10A with increasing concentrations of Calcein AM for 5 h. The data represent means±s.d. (n=3 biological replicates). The immunoblot showed the TopBP1 expression levels in these four cell lines (upper panel). (b) Cells were treated with Calcein AM (2.5 μM) overnight and then subjected to Caspase-Glo 3/7 activity assay. Shown are means±s.d. derived from three independent experiments. *P<0.001, compared with DMSO control (two-tailedt-test). (c) The effect of Calcein AM (2.5 μM) on the doxorubicin sensitivity in MCF10A and MDA-MB468 cell lines. MTS assays were performed 5 h after treatment. The 490-nm absorbance readings were normalized to the ‘0 μM Doxorubicin’ controls within each group. The MTS readings normalized to the ‘DMSO, 0 μM Doxorubicin’ control cells are presented inSupplementary Fig. 5. Shown are means±s.d. derived from three biological replicates.P<0.001 compared with DMSO control. (d) MDA-MB468 cells were seeded into an Ultra-low Adherent six-well plate with complete MammoCult medium, and then cultured for 11 days in DMSO or Calcein AM (2.5 μM). The mammospheres were observed at × 10 magnification. The diameters of 15 mammospheres were measured from three independent culture experiments using a Zeiss digital inverted microscope (Axio Observer). *P<0.001 (two-tailedt-test). Higher-magnification images are shown inSupplementary Fig. 6. (e) MDA-MB468 cells were treated with DMSO or increasing doses of Calcein AM for 16 h. Cells were then grown in fresh media without Calcein AM for eight more days and then stained with crystal violet. Each treatment was performed in triplicate. Representative images are shown in the left panels (a complete set of data are shown inSupplementary Fig. 7). Colonies were counted and colony numbers relative to DMSO controls (means±s.d.) are shown in the right graph. *P<0.001 compared with DMSO controls (two-tailedt-test). (f) In parallel with the experiment ine, some MDA-MB468 cells were treated with DMSO or increasing doses of Calcein AM for 16 h and then assayed for caspase activation. Shown are means±s.d. derived from three biological replicates. *P<0.001, compared with DMSO control (two-tailedt-test). Figure 4: Calcein AM shows antitumour activity against many different cancer cell lines. ( a ) MTS assays were performed in breast cancer cell lines MDA-MB468, MDA-MB231 and MCF7, and nontransformed breast epithelial cell line MCF10A with increasing concentrations of Calcein AM for 5 h. The data represent means±s.d. ( n =3 biological replicates). The immunoblot showed the TopBP1 expression levels in these four cell lines (upper panel). ( b ) Cells were treated with Calcein AM (2.5 μM) overnight and then subjected to Caspase-Glo 3/7 activity assay. Shown are means±s.d. derived from three independent experiments. * P <0.001, compared with DMSO control (two-tailed t -test). ( c ) The effect of Calcein AM (2.5 μM) on the doxorubicin sensitivity in MCF10A and MDA-MB468 cell lines. MTS assays were performed 5 h after treatment. The 490-nm absorbance readings were normalized to the ‘0 μM Doxorubicin’ controls within each group. The MTS readings normalized to the ‘DMSO, 0 μM Doxorubicin’ control cells are presented in Supplementary Fig. 5 . Shown are means±s.d. derived from three biological replicates. P <0.001 compared with DMSO control. ( d ) MDA-MB468 cells were seeded into an Ultra-low Adherent six-well plate with complete MammoCult medium, and then cultured for 11 days in DMSO or Calcein AM (2.5 μM). The mammospheres were observed at × 10 magnification. The diameters of 15 mammospheres were measured from three independent culture experiments using a Zeiss digital inverted microscope (Axio Observer). * P <0.001 (two-tailed t -test). Higher-magnification images are shown in Supplementary Fig. 6 . ( e ) MDA-MB468 cells were treated with DMSO or increasing doses of Calcein AM for 16 h. Cells were then grown in fresh media without Calcein AM for eight more days and then stained with crystal violet. Each treatment was performed in triplicate. Representative images are shown in the left panels (a complete set of data are shown in Supplementary Fig. 7 ). Colonies were counted and colony numbers relative to DMSO controls (means±s.d.) are shown in the right graph. * P <0.001 compared with DMSO controls (two-tailed t -test). ( f ) In parallel with the experiment in e , some MDA-MB468 cells were treated with DMSO or increasing doses of Calcein AM for 16 h and then assayed for caspase activation. Shown are means±s.d. derived from three biological replicates. * P <0.001, compared with DMSO control (two-tailed t -test). Full size image We next extended the studies to other cancer cell lines. We found that Calcein AM also inhibited the proliferation of p53-null SKOV-3 ovarian cancer cells either alone ( Fig. 5a ) or in combination with cisplatin ( Fig. 5b ). Although overexpression of mutp53(R273H) inhibited cisplatin-induced apoptosis in SKOV-3 cells (due to mutp53 GOF [19] ), this effect could be partially rescued by Calcein AM ( Fig. 5c ). Calcein AM also sensitized cells to doxorubicin in a myeloma cell line RPMI 8226 harbouring mutp53(E285K) ( Fig. 5d ). Thus, Calcein AM appears to have activity against a broad spectrum of cancer cells. In fact, Calcein AM (NSC 689290) is among the active compounds in NCI Developmental Therapeutics Program (DTP) screening programme, which utilized a panel of NCI-60 cancer cell lines to test compounds at five concentrations. The average Calcein AM GI 50 over all 60 cell lines is 0.662 μM (ranging from 10 nM to 10.96 μM, see Fig. 6a ; NCI-DTP data). The GI 50 of Calcein AM in several TNBC cell lines such as BT549 and Hs-578T, and so on, are less than 0.4 μM, and in several lung cancer cell lines such as A549, NCI-H23, NCI-H460 and NCI-H522 are less than 1 μM ( Fig. 6a ). We analysed Calcein AM sensitivity (GI 50 ) and TopBP1 RNA levels in NCI-60 cell lines from NCI-DTP server and found a correlation between high TopBP1 levels and the sensitivity Calcein AM ( r =−0.4439, two-tailed P =0.0005, Fig. 6b ). Upon examining the Akt status (in RPPA database) of those cells with discordance (that is, sensitivity does not correlate with TopBP1 expression), we found that most of them show low Akt activity (low T308 phosphorylation), for example, MDA-MB435 cells [30] ( Fig. 6a ). This suggested that the sensitivity to Calcein AM might be affected by both TopBP1 levels and Akt activity. To test this in an unbiased manner, we ranked the NCI-60 cell lines according to either pT308-Akt or total Akt levels, and calculated the Pearson correlation coefficients. While total Akt status does not affect the correlation between TopBP1 and Calcein AM sensitivity, higher pT308-Akt levels indeed show better correlation ( Fig. 6c,d ). Thus, Calcein AM has activity against a wide spectrum of cancer cells, and its sensitivity is correlated with TopBP1 levels, particularly in Akt-activated cancer cells. 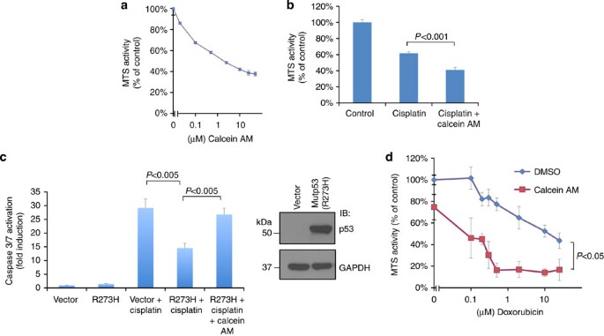Figure 5: Calcein AM sensitizes mutp53-harbouring cancer cells to chemotherapy. (a) Cell viability was measured by MTS assay in an ovarian cancer cell line SKOV-3 with increasing concentrations of Calcein AM overnight. (b) SKOV-3 cells were treated with cisplatin (20 μM) alone or with Calcein AM (5 μM) for 20 h, and then subjected to MTS assay. (c) SKOV-3 cells (p53-null) were transfected with an empty vector control or mutp53(R273H) and then treated with cisplatin (20 μM) alone or with Calcein AM (5 μM) for 20 h. Apoptosis was measured by Caspase-Glo 3/7 activity assay. Expression of mutp53 was confirmed by western blot analysis (right panel). (d) RPMI 8226 cells were treated with an increasing dose of doxorubicin along with vehicle (DMSO) or with Calcein AM (2.5 μM) for 12 h before subjecting to MTS assay. Each treatment was tested in triplicate, and the values were normalized to vehicle control wells. Results shown ina–dare means±s.d. derived from three biological replicates.Pvalues are for two-tailedt-test. Figure 5: Calcein AM sensitizes mutp53-harbouring cancer cells to chemotherapy. ( a ) Cell viability was measured by MTS assay in an ovarian cancer cell line SKOV-3 with increasing concentrations of Calcein AM overnight. ( b ) SKOV-3 cells were treated with cisplatin (20 μM) alone or with Calcein AM (5 μM) for 20 h, and then subjected to MTS assay. ( c ) SKOV-3 cells (p53-null) were transfected with an empty vector control or mutp53(R273H) and then treated with cisplatin (20 μM) alone or with Calcein AM (5 μM) for 20 h. Apoptosis was measured by Caspase-Glo 3/7 activity assay. Expression of mutp53 was confirmed by western blot analysis (right panel). ( d ) RPMI 8226 cells were treated with an increasing dose of doxorubicin along with vehicle (DMSO) or with Calcein AM (2.5 μM) for 12 h before subjecting to MTS assay. Each treatment was tested in triplicate, and the values were normalized to vehicle control wells. Results shown in a – d are means±s.d. derived from three biological replicates. P values are for two-tailed t -test. 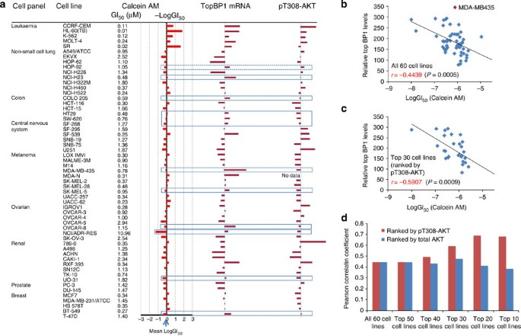Figure 6: Calcein AM sensitivity correlates with TopBP1 expression and Akt activity in NCI-60 cancer cell lines. (a) The sensitivity to Calcein AM (NSC 689290) and TopBP1 mRNA levels (GC181500) and pT308-AKT levels by RPPA (MT18349) in NCI-60 cell lines were extracted from NCI-DTP server. Box lines highlight the cell lines with discrepancy in LogGI50and TopBP1 mRNA levels. Most of the discrepancy was found in cells with low pT308-AKT levels except HOP-92 cells (dotted box). (b) The correlation between the sensitivity of NCI-60 cell lines to Calcein AM (expressed as LogGI50, the concentration that causes 50% growth inhibition) and TopBP1 RNA levels in these cell lines. Pearson correlation coefficient (r) andPvalue are shown. (c) Only the top 30 cell lines with a higher level of pT308-AKT are included in this correlative analysis. (d) The NCI-60 cell lines were ranked according to either pT308-AKT or total AKT expression levels followed by the correlative analysis with TopBP1 expression for the selected cell lines. Full size image Figure 6: Calcein AM sensitivity correlates with TopBP1 expression and Akt activity in NCI-60 cancer cell lines. ( a ) The sensitivity to Calcein AM (NSC 689290) and TopBP1 mRNA levels (GC181500) and pT308-AKT levels by RPPA (MT18349) in NCI-60 cell lines were extracted from NCI-DTP server. Box lines highlight the cell lines with discrepancy in LogGI 50 and TopBP1 mRNA levels. Most of the discrepancy was found in cells with low pT308-AKT levels except HOP-92 cells (dotted box). ( b ) The correlation between the sensitivity of NCI-60 cell lines to Calcein AM (expressed as LogGI 50 , the concentration that causes 50% growth inhibition) and TopBP1 RNA levels in these cell lines. Pearson correlation coefficient ( r ) and P value are shown. ( c ) Only the top 30 cell lines with a higher level of pT308-AKT are included in this correlative analysis. ( d ) The NCI-60 cell lines were ranked according to either pT308-AKT or total AKT expression levels followed by the correlative analysis with TopBP1 expression for the selected cell lines. Full size image E2F1 and p63/p73 mediate Calcein AM anticancer activity Since Calcein AM activates E2F1 pro-apoptotic target genes, blocks mutp53 GOF ( Fig. 3 ) and releases p73 from mutp53 binding ( Fig. 2 ), we examined whether the cytotoxic activity of Calcein AM was mediated by E2F1 and p63/p73, which were unleashed after Calcein AM interrupted TopBP1/E2F1 and TopBP1/mutp53 interactions. We chose BT549 for these studies because of their Calcein AM sensitivity and high transfection efficiency. Consistent with the low GI 50 of Calcein AM (0.27 μM, from NCI-DTP database, Fig. 6a ) for BT549 cells, Calcein AM-induced apoptosis in BT549 cells at 1 μM and above ( Fig. 7a ). Depletion of E2F1 by two short hairpin RNA (shRNA) constructs attenuated Calcein AM response as measured by caspase activation ( Fig. 7b ) and viability assay ( Fig. 7c ). Calcein AM-induced apoptosis was also decreased by depletion of p63 ( Fig. 7d ) and p73 ( Fig. 7e ). Correspondingly, there were more living cells in p63- and p73-depleted cells compared with scrambled shRNA after Calcein AM ( Fig. 7f ). Together with E2F1 and p63/p73 target gene analysis shown in Fig. 3d , these data indicate that Calcein AM activates E2F1 and p63/p73 activities to induce apoptosis. 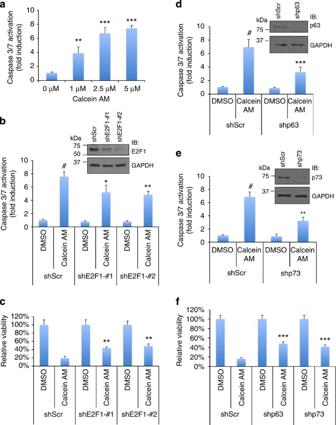Figure 7: The cytotoxicity of Calcein AM in cancer cells depends on E2F1 and p63/p73. (a) BT549 cells were treated with Calcein AM at indicated concentrations for 16 h. Apoptosis was then analysed by Caspase-Glo 3/7 activity assay. Shown are means±s.d. derived from three biological replicates. **P<0.01; ***P<0.001, compared with DMSO control (two-tailedt-test). (b) BT549 cells were transfected with two shRNAs against E2F1 or a scrambled (Scr) shRNA. Forty-eight hours after transfection, cells were treated with Calcein AM (2.5 μM) for 16 h and then subjected to Caspase-Glo 3/7 activity assay. Shown are means±s.d. derived from three biological replicates.#P<0.001 compared with DMSO group; *P<0.05; **P<0.01, compared with shScr-Calcein AM group (two-tailedt-test). Depletion of E2F1 in these samples was confirmed with western blot analysis (right panels). (c) BT549 cells were transfected with two shE2F1 as inb, and then treated with Calcein AM (2.5 μM) or DMSO for 20 h. Total number of living cells was counted with trypan blue exclusion assay and normalized to the vehicle controls. Shown are means±s.d. derived from three biological replicates. **P<0.005 compared with shScr-Calcein AM group (two-tailedt-test). (d) BT549 cells were transfected with shRNA against p63 or a scrambled (Scr) shRNA. Forty-eight hours after transfection, cells were treated with Calcein AM (2.5 μM) for 17 h and then subjected to Caspase-Glo 3/7 activity assay. Shown are means±s.d. derived from five biological replicates.#P<0.001 compared with DMSO group; ***P<0.001 compared with shScr-Calcein AM group (two-tailedt-test). Depletion of p63 was confirmed by western blot analysis (upper panels). (e) The expression of p73 in BT549 was depleted by transfecting shRNA against p73. Two days later, cells were treated with Calcein AM (2.5 μM) for 17 h and then subjected to Caspase-Glo 3/7 activity assay. Shown are means±s.d. derived from three biological replicates.#P<0.001 compared with DMSO group; **P<0.01 compared with shScr-Calcein AM group (two-tailedt-test). Depletion of p73 was confirmed by western blot analysis (upper panels). (f) BT549 cells were transfected with shp63 or shp73 as ind,e, and then treated with Calcein AM (2 μM) or DMSO vehicle for 15 h. The number of viable cells was counted by trypan blue exclusion assay and normalized to the vehicle controls. Shown are means±s.d. derived from three biological replicates. The result was replicated two times. ***P<0.001 compared with shScr-Calcein AM group (two-tailedt-test). Figure 7: The cytotoxicity of Calcein AM in cancer cells depends on E2F1 and p63/p73. ( a ) BT549 cells were treated with Calcein AM at indicated concentrations for 16 h. Apoptosis was then analysed by Caspase-Glo 3/7 activity assay. Shown are means±s.d. derived from three biological replicates. ** P <0.01; *** P <0.001, compared with DMSO control (two-tailed t -test). ( b ) BT549 cells were transfected with two shRNAs against E2F1 or a scrambled (Scr) shRNA. Forty-eight hours after transfection, cells were treated with Calcein AM (2.5 μM) for 16 h and then subjected to Caspase-Glo 3/7 activity assay. Shown are means±s.d. derived from three biological replicates. # P <0.001 compared with DMSO group; * P <0.05; ** P <0.01, compared with shScr-Calcein AM group (two-tailed t -test). Depletion of E2F1 in these samples was confirmed with western blot analysis (right panels). ( c ) BT549 cells were transfected with two shE2F1 as in b , and then treated with Calcein AM (2.5 μM) or DMSO for 20 h. Total number of living cells was counted with trypan blue exclusion assay and normalized to the vehicle controls. Shown are means±s.d. derived from three biological replicates. ** P <0.005 compared with shScr-Calcein AM group (two-tailed t -test). ( d ) BT549 cells were transfected with shRNA against p63 or a scrambled (Scr) shRNA. Forty-eight hours after transfection, cells were treated with Calcein AM (2.5 μM) for 17 h and then subjected to Caspase-Glo 3/7 activity assay. Shown are means±s.d. derived from five biological replicates. # P <0.001 compared with DMSO group; *** P <0.001 compared with shScr-Calcein AM group (two-tailed t -test). Depletion of p63 was confirmed by western blot analysis (upper panels). ( e ) The expression of p73 in BT549 was depleted by transfecting shRNA against p73. Two days later, cells were treated with Calcein AM (2.5 μM) for 17 h and then subjected to Caspase-Glo 3/7 activity assay. Shown are means±s.d. derived from three biological replicates. # P <0.001 compared with DMSO group; ** P <0.01 compared with shScr-Calcein AM group (two-tailed t -test). Depletion of p73 was confirmed by western blot analysis (upper panels). ( f ) BT549 cells were transfected with shp63 or shp73 as in d , e , and then treated with Calcein AM (2 μM) or DMSO vehicle for 15 h. The number of viable cells was counted by trypan blue exclusion assay and normalized to the vehicle controls. Shown are means±s.d. derived from three biological replicates. The result was replicated two times. *** P <0.001 compared with shScr-Calcein AM group (two-tailed t -test). Full size image A novel TopBP1-dependent mechanism for Calcein AM activity With the correlation between TopBP1 levels and Calcein AM sensitivity in NCI-60 cancer cell lines ( Fig. 6 ), we investigated how TopBP1 levels affected Calcein AM response. Overexpression of TopBP1 in MDA-MB231 cells that express TopBP1 at lower levels rendered cells more resistant to doxorubicin. This result demonstrates the activity of TopBP1 in repressing doxorubicin-induced apoptosis. Importantly, this anti-apoptotic activity of TopBP1 was blocked by Calcein AM ( Fig. 8a and Supplementary Fig. 8a ). On the other hand, consistent with previous data on the upregulation of E2F1- and p63/p73-dependent pro-apoptotic target gene expression by TopBP1 knockdown [9] , [19] , TopBP1 depletion sensitized MDA-MB468 to doxorubicin treatment ( Fig. 8b and Supplementary Fig. 8b ). While Calcein AM sensitized the shScr control MDA-MB468 cells to doxorubicin, it failed to cast the same effect on TopBP1-depleted MDA-MB468 cells ( Fig. 8b and Supplementary Fig. 8b ). Acute depletion of TopBP1 in HEK293 cells induced E2F1-dependent apoptosis [8] . Calcein AM also induced apoptosis in HEK293 cells ( Fig. 8c ). In the TopBP1-depleted HEK293 cells where E2F1 activity has been unleashed, Calcein AM could not induce more apoptosis ( Fig. 8c ). The data in Fig. 8a–c indicate that Calcein AM blocks TopBP1 anti-apoptotic activity and that Calcein AM and TopBP1 shRNAs were targeting the same molecules or pathways. Together with the analysis of NCI-60 cell lines in Fig. 6 , these data support TopBP1 as an in vivo target for Calcein AM. To rule out the possibility that Calcein AM might cause DNA damage through other undefined mechanisms, we treated MDA-MB468 with this compound up to 10 μM and still did not see evidence of DNA damage as shown by lack of either pS15-p53 or γ-H2AX signal ( Supplementary Fig. 9 ). We also examined whether Calcein AM might interfere with TopBP1 checkpoint activation. In fact, Calcein AM did not block hydroxyurea-induced Chk1 activation ( Supplementary Fig. 10 ), and might slightly promote Chk1 activation in a TopBP1-dependent manner. This is consistent with the effect of Calcein AM in blocking TopBP1 oligomerization and shifting TopBP1 towards monomeric form for checkpoint activation. Taken together, Calcein AM selectively kills cancer cells through a TopBP1-dependent mechanism of action. 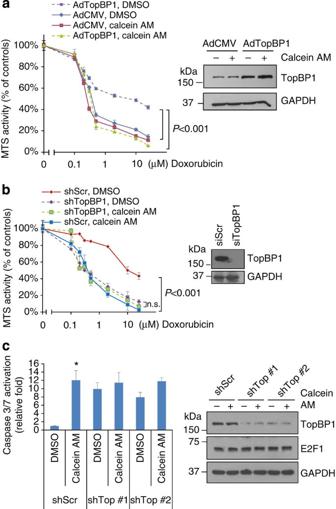Figure 8: The sensitivity to Calcein AM in cancer cells depends on TopBP1. (a) MDA-MB231 cells were infected with recombinant adenoviruses expressing empty vector (AdCMV) or AdTopBP1 (multiplicity of infection 500). After 2 days, the sensitivity to doxorubicin in the presence of DMSO or Calcein AM (2.5 μM) was measured as inFig. 4c. Shown are means±s.d. from three biological replicates. TopBP1 overexpression was confirmed by western blotting (right panel). The 490-nm absorbance readings were normalized to the ‘0 μM Doxorubicin’ controls within each group. The MTS readings normalized to the ‘DMSO, 0 μM Doxorubicin’ control cells are presented inSupplementary Fig. 8a. (b) Doxorubicin sensitivity was assayed in TopBP1-depleted MDA-MB468 cells treated with doxorubicin and either DMSO or Calcein AM (2.5 μM) for 5 h and then subjected to MTS assay. Shown are means±s.d. from three biological replicates. TopBP1 knockdown was confirmed by western blotting (right panel). n.s.: not significant. The MTS readings are relative to the ‘0 μM Doxorubicin’ controls of each group. The MTS readings normalized to the ‘DMSO, 0 μM Doxorubicin’ control cells are presented inSupplementary Fig. 8b. (c) HEK293 cells transfected with pSuper-shScr or two different pSuper-shTopBP1 constructs (shTop no. 1 and no. 2)8were treated with 2.5 μM Calcein or DMSO overnight. Apoptosis was measured by Caspase-Glo 3/7 activity assay. *P=0.001, compared with shScr control group (two-tailedt-test,n=3 biological replicates). E2F1 expression and depletion of TopBP1 were shown by immunoblotting (right panel). Figure 8: The sensitivity to Calcein AM in cancer cells depends on TopBP1. ( a ) MDA-MB231 cells were infected with recombinant adenoviruses expressing empty vector (AdCMV) or AdTopBP1 (multiplicity of infection 500). After 2 days, the sensitivity to doxorubicin in the presence of DMSO or Calcein AM (2.5 μM) was measured as in Fig. 4c . Shown are means±s.d. from three biological replicates. TopBP1 overexpression was confirmed by western blotting (right panel). The 490-nm absorbance readings were normalized to the ‘0 μM Doxorubicin’ controls within each group. The MTS readings normalized to the ‘DMSO, 0 μM Doxorubicin’ control cells are presented in Supplementary Fig. 8a . ( b ) Doxorubicin sensitivity was assayed in TopBP1-depleted MDA-MB468 cells treated with doxorubicin and either DMSO or Calcein AM (2.5 μM) for 5 h and then subjected to MTS assay. Shown are means±s.d. from three biological replicates. TopBP1 knockdown was confirmed by western blotting (right panel). n.s. : not significant. The MTS readings are relative to the ‘0 μM Doxorubicin’ controls of each group. The MTS readings normalized to the ‘DMSO, 0 μM Doxorubicin’ control cells are presented in Supplementary Fig. 8b . ( c ) HEK293 cells transfected with pSuper-shScr or two different pSuper-shTopBP1 constructs (shTop no. 1 and no. 2) [8] were treated with 2.5 μM Calcein or DMSO overnight. Apoptosis was measured by Caspase-Glo 3/7 activity assay. * P =0.001, compared with shScr control group (two-tailed t -test, n =3 biological replicates). E2F1 expression and depletion of TopBP1 were shown by immunoblotting (right panel). Full size image Calcein AM inhibits the growth of breast cancer xenografts To investigate the in vivo activity of Calcein AM, we next established MDA-MB468 xenografts in nude mice and injected intraperitoneally (i.p.) with Calcein AM (40 mg kg −1 ) or vehicle (dimethylsulphoxide (DMSO)) every 3 days for three doses (five mice per group). Two independent experiments showed that Calcein AM significantly inhibited xenograft growth ( Fig. 9a,b and Supplementary Fig. 11 ) as well as the expression of proliferation marker Ki-67 ( Supplementary Figs 12 and 13 ) without affecting body weights of mice ( Fig. 9c and Supplementary Fig. 11c ). When the tumours started to regrow around day 60 in the experiment of Supplementary Fig. 11 , a second round of treatment was given on day 61 since. The tumours responded to Calcein AM injection again. Immunohistochemistry (IHC) of the xenografts harvested 1 week after the second injection showed inhibition of proliferation and induction of apoptosis, as indicated by Ki-67 staining, TdT-mediated dUTP nick end labeling (TUNEL) assay and cleaved caspase 3 staining ( Fig. 9d ). 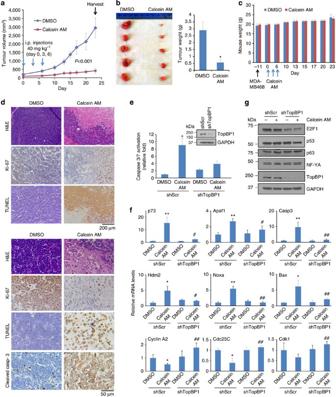Figure 9: Effect of Calcein AM on tumour growth in the MDA-MB468 xenograft model and impact of TopBP1 on Calcein AM response in cultured MDA-MB468 cells. (a) Nude mice bearing MDA-MB468 xenografts were administered with Calcein AM or vehicle DMSO via i.p. injection. The mean tumour volumes±s.d. are shown;n=5 mice per group. This result was replicated and shown inSupplementary Fig. 11. (b) Photographs of the MDA-MB468 xenograft tumours (left) and tumour weights (right)). *P<0.001 (two-tailedt-test). (c) The mean mouse body weights±s.d. (n=5) from the injection of MDA-MB468 cells (day −11). (d) Representative images of haematoxylin and eosine (H&E), Ki-67, immunohistochemical staining and TUNEL staining of xenografts at × 10 magnification (upper panels). Representative images of H&E, Ki-67, TUNEL and cleaved caspase 3 staining at × 40 magnification (lower panels). (e) The effect of Calcein AM in MDA-MB468 cells depended on TopBP1. TopBP1-depleted MDA-MB468 cells were treated with Calcein AM (2.5 μM) overnight and then subjected to Caspase-Glo 3/7 activity assay. siScr: scrambled RNAi control. *P=0.002, compared with siScr/DMSO,P=0.01 compared with siTopBP1/Calcein AM (two-tailedt-test,n=3). Depletion of TopBP1 was verified by western blot analysis (upper panel). (f) TopBP1-depleted and the siScr control MDA-MB468 cells were treated with Calcein AM (2.5 μM, 5 h), and E2F1, p53 and NF-Y target gene expression was analysed with qRT–PCR as inFig. 3d. **P<0.01, *P<0.05, compared with DMSO samples;##P<0.01,#P<0.05, compared with siScr/Calcein AM samples (two-tailedt-test). The data represent means±s.d. (n=3). (g) Aliquots of the cell lysates infwere analysed for western blotting. Figure 9: Effect of Calcein AM on tumour growth in the MDA-MB468 xenograft model and impact of TopBP1 on Calcein AM response in cultured MDA-MB468 cells. ( a ) Nude mice bearing MDA-MB468 xenografts were administered with Calcein AM or vehicle DMSO via i.p. injection. The mean tumour volumes±s.d. are shown; n =5 mice per group. This result was replicated and shown in Supplementary Fig. 11 . ( b ) Photographs of the MDA-MB468 xenograft tumours (left) and tumour weights (right)). * P <0.001 (two-tailed t -test). ( c ) The mean mouse body weights±s.d. ( n =5) from the injection of MDA-MB468 cells (day −11). ( d ) Representative images of haematoxylin and eosine (H&E), Ki-67, immunohistochemical staining and TUNEL staining of xenografts at × 10 magnification (upper panels). Representative images of H&E, Ki-67, TUNEL and cleaved caspase 3 staining at × 40 magnification (lower panels). ( e ) The effect of Calcein AM in MDA-MB468 cells depended on TopBP1. TopBP1-depleted MDA-MB468 cells were treated with Calcein AM (2.5 μM) overnight and then subjected to Caspase-Glo 3/7 activity assay. siScr: scrambled RNAi control. * P =0.002, compared with siScr/DMSO, P =0.01 compared with siTopBP1/Calcein AM (two-tailed t -test, n =3). Depletion of TopBP1 was verified by western blot analysis (upper panel). ( f ) TopBP1-depleted and the siScr control MDA-MB468 cells were treated with Calcein AM (2.5 μM, 5 h), and E2F1, p53 and NF-Y target gene expression was analysed with qRT–PCR as in Fig. 3d . ** P <0.01, * P <0.05, compared with DMSO samples; ## P <0.01, # P <0.05, compared with siScr/Calcein AM samples (two-tailed t -test). The data represent means±s.d. ( n =3). ( g ) Aliquots of the cell lysates in f were analysed for western blotting. Full size image We also tested the in vivo activity of Calcein AM against the xenograft formation in another cell line BT549. Twenty nude mice were injected subcutaneously (s.c.) with BT549 cells. Four days later, mice were then injected i.p. either with DMSO (eight mice), Calcein AM 20 mg kg −1 (eight mice) or Calcein AM 40 mg kg −1 (four mice) every 3 days for three doses. Six out of eight DMSO-treated mice developed xenografts later. On the contrary, none of the eight mice injected with Calcein AM 20 mg kg −1 and none of the four mice injected with Calcein AM 40 mg kg −1 developed tumours ( Supplementary Fig. 14 ). Thus, Calcein AM has in vivo activity against tumour growth or development in MDA-MB468 and BT549 xenograft models. The mice appeared to tolerate Calcein AM i.p. injections throughout the course of treatment. To investigate whether there was any acute toxicity in proliferating tissues, we injected Calcein AM 40 mg kg −1 and analysed intestinal tissues 48 h after injection. As shown in Supplementary Fig. 15 , Calcein AM injection did not decrease Ki-67 staining, nor did it induce apoptosis in the intestinal epithelium. The lack of toxicity in normal mouse tissues could be in principle because of a species-specific activity of Calcein AM against human cells, but not mouse cells. However, this is unlikely, since TopBP1-BRCT7/8 is highly conserved between human and mouse (74% identify, 83.3% similarity), and the predicted calcein contact residues K1317, R1280, S1273, S1274, R1314 and R1407 ( Fig. 1e ) are 100% conserved in mouse TopBP1. To rule out this possibility, we tested the activity of Calcein AM in mouse and rat tumour cells. As shown in Supplementary Fig. 16 , Calcein AM also induced apoptosis in mouse breast tumour cells 4T1 and rat hepatoma cells McA-RH7777. Thus, Calcein AM selectively kills cancer cells but is not toxic to normal tissues. We further utilized the MDA-MB468 cells expressing shTopBP1 to validate the in vivo target of Calcein AM. Indeed, depletion of TopBP1 mitigated the effect of Calcein AM on apoptosis ( Fig. 9e ; the results were reproduced in Supplementary Fig. 17 using two different shTopBP1). Correspondingly, the induction of E2F1, p63/p73 and NF-Y target gene expression by Calcein AM treatment was less significant in these TopBP1-depleted cells ( Fig. 9f ). We noted that in the TopBP1-depleted MDA-MB468 cells, E2F1 levels were reduced ( Fig. 9g and Supplementary Fig. 17 ). It is possible that acute depletion of TopBP1 induces E2F1-dependent apoptosis [8] ; thus, high E2F1-expressing cells would be counterselected, resulting in selecting for the cells with lower E2F1 expression. To investigate the role for E2F1 in mediating the effect of TopBP1 depletion, we carried out doxycycline-inducible depletion of TopBP1 or both TopBP1 and E2F1 in U2OS cells ( Fig. 10a ) using the U2OS T-REX system [12] , [31] , [32] . The results show that upon depletion of TopBP1 after adding doxycycline (to induce TopBP1 shRNA), there was a decrease in cell number. This was a reversible and likely regulatory effect by TopBP1, since the defect was immediately rescued by restoring TopBP1 expression upon withdrawal of doxycycline. Thus, it is unlikely because of structural genomic damage from TopBP1 depletion. Importantly, the reduction in cell number by TopBP1 depletion was largely rescued upon concurrent depletion of E2F1 ( Fig. 10a ). This result indicates that the role of TopBP1 in cell proliferation/apoptosis is in part mediated through its regulation on E2F1. Therefore, Calcein AM sensitivity is affected by TopBP1 and E2F1 levels in cancer cells. 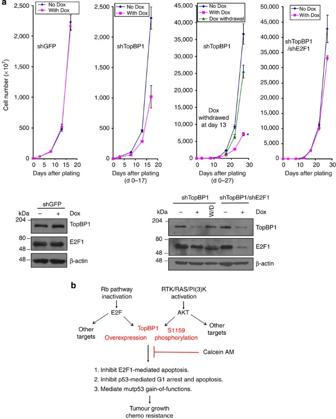Figure 10: Role of E2F1 in mediating growth suppression upon TopBP1 depletion and a scheme summarizing the present studies. (a) The decrease in cell number upon TopBP1 depletion is in part dependent on E2F1. We first established U2OS stable cell lines for doxycycline-inducible expression of control shGFP, shTopBP1 and both shTopBP1 and shE2F1 using the T-REX system12,31,32. ShRNAs were then induced with doxycycline (DOX) on day 0 (pink lines), and cells were counted using a Beckman Coulter counter. An aliquot of DOX-treated shTopBP1 cells were plated in medium without Dox (Dox withdrawal, W/D) since day 13 (third graph from the left, Dox withdrawal, green line). To make it easy to compare, day 0–17 of shTopBP1 was plotted (second graph from the left) for comparison with shGFP, and day 0–27 of shTopBP1 was plotted (third graph from the left) for comparison with shTopBP1/shE2F1. The data represent means±s.d. from three biological replicates. *P<0.001 when compared with ‘no Dox’, andP<0.01 when compared with ‘Dox withdrawal’ (two-tailedt-test). Lower panels: western blots of TopBP1 and E2F1. (b) TopBP1 is at a convergent point between Rb and PI(3)K signalling pathways and contributes to tumour progression through E2F1 and p53 regulation. Its action is blocked by Calcein AM. Figure 10: Role of E2F1 in mediating growth suppression upon TopBP1 depletion and a scheme summarizing the present studies. ( a ) The decrease in cell number upon TopBP1 depletion is in part dependent on E2F1. We first established U2OS stable cell lines for doxycycline-inducible expression of control shGFP, shTopBP1 and both shTopBP1 and shE2F1 using the T-REX system [12] , [31] , [32] . ShRNAs were then induced with doxycycline (DOX) on day 0 (pink lines), and cells were counted using a Beckman Coulter counter. An aliquot of DOX-treated shTopBP1 cells were plated in medium without Dox (Dox withdrawal, W/D) since day 13 (third graph from the left, Dox withdrawal, green line). To make it easy to compare, day 0–17 of shTopBP1 was plotted (second graph from the left) for comparison with shGFP, and day 0–27 of shTopBP1 was plotted (third graph from the left) for comparison with shTopBP1/shE2F1. The data represent means±s.d. from three biological replicates. * P <0.001 when compared with ‘no Dox’, and P <0.01 when compared with ‘Dox withdrawal’ (two-tailed t -test). Lower panels: western blots of TopBP1 and E2F1. ( b ) TopBP1 is at a convergent point between Rb and PI(3)K signalling pathways and contributes to tumour progression through E2F1 and p53 regulation. Its action is blocked by Calcein AM. Full size image Taken together, Calcein AM targets TopBP1/E2F1 and TopBP1/mutp53 interactions and exerts its in vivo antitumour activity. We identify a lead compound targeting C-terminal BRCT domains of TopBP1 and provide proof-of-concept evidence to support TopBP1 as a novel cancer therapeutic target that functions in a convergent point of multiple oncogenic pathways: inactivation of the Rb pathway leads to its overexpression, and activation of RTK/RAS/PI(3)K induces its phosphorylation. The accumulation of phosphorylated TopBP1 in cancer cells may cause defects in growth checkpoints through repressing E2F1 and p53 functions, and turning mutp53 into oncoproteins ( Fig. 10b ). Using a small molecule inhibitor capable of blocking the endogenous interactions between TopBP1 and E2F1 as well as mutp53, we validate TopBP1 as a therapeutic target in the tumours to activate E2F1 pro-apoptotic activity and to avert the oncogenic activity of mutp53. While the cytotoxic activity of Calcein AM against cancer cells was noticed before, we now identify its in vivo target and elucidate its selective antitumour activity through a novel TopBP1-dependent mechanism of action. Finally, for the first time we demonstrate Calcein AM antitumour activity in two breast cancer xenograft models. While drug development typically aims at upstream receptors/kinases, our study provides evidence for targeting the proteins in the nexus of multiple signalling pathways as new cancer therapeutics. Different mutant p53 proteins may have different functions. TopBP1 can bind to several hot spot mutants, including both DNA contact mutant (such as R273H) and conformational mutants (such as R175H and R249S) [19] . Consistently, by targeting TopBP1, Calcein AM releases p73 from mutp53(R273H) in MDA-MB468 cells and from mutp53(R249S) in BT549 cells. Although the effect of Calcein AM against each mutant p53 will need to be tested experimentally, the two examples presented here suggest that Calcein AM might be used to treat cancer cells harbouring a broad spectrum of p53 mutations. In BT549 cells, we demonstrated a role for E2F1 and p63/p73 for mediating Calcein AM-induced apoptosis ( Fig. 7 ). TopBP1-BRCT7/8 also binds to other transcription factors, such as Miz1 (refs 9 , 33 ). In fact, Calcein AM treatment also released Miz1 from TopBP1 ( Fig. 2f ), suggesting that Miz1 might also contribute to the toxic effects of Calcein AM. The other factor worth considering is the difference in genetic alterations causing Akt activation in cancer. PTEN loss mainly occurs in basal-like breast cancer, whereas PIK3CA mutations are more common in luminal or Her2E subtype breast cancer [1] . Both MDA-MB468 and BT549 cell lines tested here have PTEN loss. Whether cancer cells with PIK3CA mutations respond differently to Calcein AM will be tested in the future. According to NCI-60 cell line database, a PIK3CA mutant (H1049R) cell line T47D still responds to Calcein AM (GI 50 1.4 μM; Fig. 6a ). Calcein AM has been considered to be nontoxic to a wide spectrum of cell types especially in normal cells and thus is widely used for viability assay and in vivo physiological cell marking. The fact that the mice injected with Calcein AM did not manifest any apparent toxicity in our study indicates that the dose (40 mg kg −1 ) that is effective in shrinking MDA-MB468 xenografts is quite tolerable for the mice. Consistently, the toxicology study of Calcein AM performed by Dojindo Laboratories shows that oral LD50 in rats is 14.5 g kg −1 ; oral LD50 in mice is 17 g kg −1 ; percutaneous LD50 in mice is 5 g kg −1 (according to Material Safety Data Sheet, http://www.dojindo.com/store/p/162-Cellstain-Calcein-AM-Solution.html ). On the other hand, calcein may bind ions such as Ca and Mg; thus, the potential effects of ion chelation need to be considered. However, it only binds these ions at strong alkaline pH (therefore, it is now rarely used as intracellular Ca indicator). A more potent intracellular calcium chelator BAPTA/AM in fact has a neuroprotective effect by preventing the cell damage caused by elevated cytoplasmic Ca levels [34] during cerebral ischaemia. Moreover, the cytotoxicity of Calcein AM in cancer cells that we observed depends on TopBP1, and Calcein AM treatment induces E2F1 and mutp53 target gene changes. Thus, it is unlikely that the cytotoxicity is caused by calcium chelation. Another potential property of Calcein AM that warrants consideration is its sensitivity to reactive oxygen species (ROS). After removal of the acetomethoxy side chain, calcein can be oxidized and it becomes fluorescent. Thus, it was proposed to be used as a detector of intracellular oxidative activity [35] . However, the ROS-sensitive fluorescein derivatives do not produce oxidative damage (instead they recycle ROS) and, therefore, are used to detect intracellular ROS generation in living cells (Molecular Probes). Lack of pS15-p53 signal after Calcein AM treatment ( Supplementary Fig. 9 ) also indicates that it does not produce oxidative damage or DNA damage. TopBP1 protein is overexpressed in nearly 60% (46 out of 79 cases) of primary breast cancer tissues when compared with matched uninvolved breast tissues using western blot and IHC analyses [12] . An increased risk of breast cancer relapse or death is seen in patients with tumours containing high levels of TopBP1 protein [12] or TopBP1 RNA (analysis of four breast databases composed of 1,028 patients [19] ). Activation of PI(3)K/Akt signalling occurs in 77% of breast cancer [1] . Thus, this convergent event is expected to be quite prevalent in breast cancer, particularly in TNBCs that overexpress TopBP1 in nearly all cases [12] and harbour mutp53 in 84% of cases [1] . Therefore, the impact of this novel therapy would be very significant for many breast cancer patients. Moreover, these oncogenic pathways are common to many cancers. For example, the genetic alterations in glioblastoma occur mainly in these three signalling pathways: RTK/RAS/PI(3)K (88%), p53 (87%) and Rb (78%) [36] . Mutations in p53 and PI3K/Akt pathways are among the most frequent genetic abnormalities in all cancers and are strongly associated with poor prognosis, and resistance to therapy. Hence, the anti-TopBP1 therapy might be applicable to many other types of cancer. Cell culture and transfection Human embryonic kidney cell lines HEK293 and HEK293T, human breast cancer cell lines MDA-MB468, MDA-MB231 and MCF7, human ovarian cancer cell line SKOV-3, human non-small cell lung cancer cell line NCI-H1299, mouse mammary carcinoma cell line 4T1 and rat hepatoma cell line McA-RH7777 were maintained in DMEM with 10% fetal bovine serum (FBS). MCF10A, a normal human breast epithelial cell line, was maintained in DMEM/F12 with 5% horse serum, 2.5 mM glutamine, 0.5 μg ml −1 hydrocortisone, 10 μg ml −1 insulin, 100 ng ml −1 cholera toxin and 20 ng ml −1 epidermal growth factor. Human breast cancer cell line BT549 and human myeloma cell line RPMI 8226 cells were maintained in RPMI with 10% FBS. All cell lines were obtained from ATCC and were tested negative for mycoplasma contamination. For maintenance, all cell lines were kept in 37 °C humidified incubator with 5% CO 2 . For HEK293, HEK293T and NCI-H1299 cells, standard calcium phosphate method was used for transfection. Polyethylenimine was used to transfect MDA-MB468 cells and in some experiments of HEK293T cells. SKOV-3 cells were transfected by electroporation (Bio-Rad). BT549 cells were transfected using the Gene Pulser Xcell Electroporation System or polyethylenimine. Virtual screening and docking Schrödinger suite (version 2010, Schrödinger, LLC, New York, NY, 2010), which includes all of the programmes described below, was used to carry out molecular modelling and docking studies. TopBP1-BRCT7/8 protein (PDB code: 3AL3) was prepared using the protein preparation wizard in Maestro 9.1 with default protein parameters: water molecules were removed, hydrogen atoms added and the BACH1 peptide ligand extracted for docking. H-bonds were optimized and the protein was energetically minimized using OPLS2005 force field. A receptor grid, which is large enough to contain the whole active site, was generated using the programme Glide without constraints. In all, 2,000 compounds from Microsource Spectrum Collection were used for the virtual screening. Compound structures were prepared using the programme LigPrep and then docked into the protein using Glide (docking parameters: standard precision and dock flexibly). The top 100 compounds were analysed manually, among which 61 compounds with M.W. greater than 250 were purchased from commercial vendors for further testing. In vitro peptide binding The GST fusion proteins in Escherichia coli strain BL21 were induced by 0.1 mM isopropyl-β-D-thiogalactopyranoside and purified according to the standard protocol. The GST portion on GST-TopBP1-BRCT7/8 was excised by Pre-Scission protease (Pharmacia). Two purified (>98%) biotin-conjugated peptides were synthesized from Sigma Genosys. The peptide sequence is derived from the surrounding sequence of TopBP1 S1159: phosphorylated peptide, Btn-REERARLApSer 1159 NLQWPS and nonphosphorylated peptide, Btn-REERARLASNLQWPS. Purified TopBP1-BRCT7/8 (2 μg) was incubated with compounds in NETN-A buffer (50 mM NaCl, 1 mM EDTA, 20 mM Tris, 0.5% NP-40) at 4 °C for 3 h with constant rotation. Then, 2 μg of purified phosphorylated peptide or nonphosphorylated peptides were added and rotated for another 3 h at 4 °C. The biotin-conjugated peptides were then pulled down with streptavidin Sepharose (Amersham). The beads were washed six times with NETN-B buffer (100 mM NaCl, 1 mM EDTA, 0.2 mM phenylmethylsulfonyl fluoride) and then subjected to sodium dodecyl sulfate–polyacrylamide gel electrophoresis (SDS–PAGE) and analysed by western blotting with anti-TopBP1 antibody (1:1,000, BL893, Bethyl Laboratories). GST pull-down assay Purified TopBP1-BRCT7/8 (2 μg) was incubated with compounds in NETN-A buffer as above at 4 °C for 3 h with constant rotation. Then purified GST-p53-DBD or GST (2 μg) were added and rotated for another 3 h at 4 °C. GST-p53-DBD was then pulled down with glutathione-Sepharose. The beads were washed six times with NETN-B buffer and then subjected to SDS–PAGE analysis. Immunoprecipitation and western blot analysis MDA-MB468 cells were lysed with TNN buffer [7] . An aliquot of cell lysates was lysed with SDS lysis buffer and the rest of cell lysates were incubated with appropriate antibodies or beads at 4 °C for 3–12 h. Anti-FLAG beads (Sigma) were washed three times with TNN buffer. Immunoprecipitates were fractionated by SDS–PAGE and electrotransferred to an Immobilon-P membrane (Millipore). Equal amount of protein loading was validated with Ponceau-S staining. The specific signals were detected by incubating with appropriate antibody. All primary antibodies were used at 1:1,000 dilution and horseradish peroxidase-conjugated secondary antibodies were used at 1:5,000 dilution for immunoblotting. E2F1 (C-20 and KH-95), p53 (FL393), p63 (4A4 and H-129), p73 (H-79), p21 (C-19), Bax (N-20), GST (B-14), c-Myc (A14), Miz1 (H-190), Chk1 (G4), Actin (C-2) and Glyceraldehyde-3-phosphate dehydrogenase (GAPDH) (6C5) antibodies were purchased from Santa Cruz. TopBP1 (mouse monoclonal) and Akt antibodies were purchased from BD Transduction Laboratories. TopBP1 (BL893, Rabbit polyclonal) antibody was purchased from Bethyl. Mouse monoclonal anti-phospho-γH2AX was purchased from Millipore. Phospho-Chk1 (Ser345) antibody was purchased from Cell signaling. FLAG (F7425) antibody was purchased from Sigma. Mouse monoclonal anti-p73 (IMG-246) was purchased from IMGENEX. Full blots are shown in Supplementary Fig. 19 . Crosslinking Borate buffer (50 mM NaBorate, 100 mM potassium acetate, 2 mM MgCl 2 , 1 mM EGTA, 1% Trition X-100 and protease inhibitors (pH 8.57)) was used to lyse MDA-MB468 cells on ice for 10 min, followed by 10-min high-speed centrifugation to remove insoluble material, and then incubated with 20 mM freshly prepared DMP (Thermo Scientific) for 30 min. An equal volume of 50 mM NH 4 Cl in PBS was added and incubated for 10 min to stop the reaction. The cell lysates were subjected to SDS–PAGE and western blot analysis. Luciferase assay E2F1 activity reporter assay using a p14 ARF promoter-luciferase plasmid was performed as described [7] . p53 activity reporter assay was performed by a p21 Cip promoter-luciferase plasmid [12] . p73 activity reporter assay was performed using a pGL3-Bax promoter-luciferase plasmid [19] . pRL-TK (Renilla luciferase, Promega) was used in all experiments for controlling transfection efficiency. The firefly and Renilla luciferase activities were measured with the Dual-Luciferase Reporter System (Promega), and the firefly luciferase activities were normalized against the Renilla activity. All assays were performed in triplicate. Real-time RT–PCR RNA was isolated using the TRIzol method (Invitrogen). Quantitative reverse transcription–PCR (RT–PCR) was performed in triplicate using the forward and reverse primers ( Supplementary Fig. 18 ) on an MX3005P thermal cycler using the SYBR green dye method to observe the progress of the reactions with ROX dye, which was added as reference. GAPDH was run in parallel with target genes. MTS assay Cells (10 4 cells per well) were plated into 48-well plates (BD Falcon) and treated with DMSO or Calcein AM separately. Then, 50 μl of MTS reagent (CellTiter 96 AQueous One Solution Cell Proliferation Assay, Promega) was added to each well, covered from light and incubated for 1 h at 37 °C incubator to develop purple colour. The samples were measured at 490 nm in a plate reader (BioTek Synergy HT) against a blank 48-well plate. Each assay was conducted in triplicate. Caspase 3/7 activation assay The apoptosis was measured by Caspase-Glo 3/7 assay (Promega) following the manufacturer’s protocol. The cells were plated in six-well tissue culture dish (10 4 cells per well; BD Falcon) in respective media. Next day, the cells were treated with DMSO (as negative control) and Calcein AM for 5 h. The blank reactions were prepared per direction. Equal volume of Caspase-Glo 3/7 reagents were applied to each well. A luminometer (Sirius) was used to quantitate luminescence. Colony formation assay MDA-MB468 cells were plated in six-well plates at 200 cells per well. The cells were either treated with DMSO vehicle or with indicated concentration of Calcein AM for 16 h and then released by three times 1 × PBS washing. Cells were grown in fresh media without drugs for additional 8 days to form colonies, when each colony contained more than 50 cells. Plates were then stained with 5% crystal violet (0.5 g crystal violet, 25 ml methanol and 75 ml H 2 O). Cell number was counted. Mammosphere formation and treatment For in vitro mammosphere culture, ~5,000 MDA-MB468 cells per well were seeded into a Ultra-low Adherent six-well plate (Stem Cell Technologies) with 2 ml per well fresh complete MammoCult medium (Stem Cell Technologies) containing the MammoCult Basal Medium, MammoCult Proliferation Supplement, 4 μg ml −1 Heparin (Stem Cell Technologies) and fresh 0.48 μg ml −1 Hydrocortisone. Cells were incubated in a 5% CO 2 incubator at 37 °C for 7–11 days. Both the untreated (DMSO-treated) and Calcein AM-treated mammospheres were observed at × 10 magnification and measured on day 11 under a Zeiss digital Axio Observer inverted microscope. Each treatment was carried out in triplicate. Gene knockdown To prepare TopBP1 knockdown stable cell line, MDA-MB468 cells were infected with lentivirus expressing TopBP1 shRNA [19] as well as scramble shRNA, separately. The infected cells were grown for 48 h followed by selection with puromycin (2 μg ml −1 ). After selection, the knockdown was confirmed by western blotting before further experiments. Two different pLKO-shTopBP1 (no. 1 and no. 2) constructs (Open Biosystems, RHS4533-NM_007027) were used to deplete TopBP1 in MDA-MB468 cells. Additional two pSuper-shTopBP1 constructs [8] were used to knock down TopBP1 in HEK293 cells. Two pSuper-shE2F1 constructs were used to deplete E2F1: shE2F1 no. 1 (described prevously [8] ), and shE2F1 no. 2 (target sequence 5′-GACTGTGACTTTGGGGACC-3′). The target sequence for pSuperior-shE2F1 is the same as pSuper-shE2F1 no. 1. To deplete p63, shp63alpha pLKO.1-puro (from Addgene, 19120) was used. TP73 MISSION shRNA (shp73 pLKO.1-puro) was purchased from Sigma (TRCN00002722587). Xenograft experiment Female nu / nu mice (4–5 weeks old) were purchased from Charles River Laboratories (Cambridge, MA, USA). The animals were cared for and maintained by the Animal Care and Use Committee of Baylor College of Medicine. Freshly grown MDA-MB468 breast cancer cells ((8 × 10 6 ) cells per site in 100 μl PBS) were injected subcutaneously into the right side of the flank of the 5- to 6-week-old mice. When tumours were measureable, the mice were randomly divided into treatment and control groups. Calcein AM was dissolved in DMSO and was given intraperitoneally at 40 mg kg −1 for three doses every third day. The control group mice were injected with vehicle (DMSO) in the same way. The mice were monitored thrice per week. The weight of the mice and tumour size were measured on the indicated day with a caliper and calculated based on the formula π /6 (length × depth × width). The evaluator was blinded to the group allocation during monitoring. Animals were killed in the indicated dates, and tumours were harvested, weighed and further processed for histopathological analysis. All experiments were performed under a Baylor College of Medicine Institutional Animal Care and Use Committee (IACUC)-approved protocol and all experiments confirm to IACUC standards and ethical regulations. Histology and IHC Both control (DMSO) and Calcein AM-treated tumour samples were placed in cassettes and fixed in 10% neutral buffered formalin overnight. Next day, the samples were sent to The Pathology and Histology Core of Baylor College of Medicine for further processing. The paraffin-embedded sections were stained with haematoxylin and eosine, Ki-67, TUNEL and anti-cleaved caspase 3 using standard operating protocols. Statistical analyses We performed two-tailed t -test for comparisons of treatment groups. P values less than 0.05 were considered statistically significant. Pearson correlation coefficient was calculated to evaluate correlations between the mRNA expression of TopBP1 and LogGI 50 of Calcein AM in NCI-60 cell lines. The sample size of the xenograft study was chosen to detect 50% response rate of xenografts, and use 5% for type II error (5% chance false negative, i.e. the number of animals to allow a 95% chance to detect an effect), then n =log 0.05/log 0.5=4.3. Thus, using five animals per group will have greater than 95% of statistical power. How to cite this article: Chowdhury, P. et al. Targeting TopBP1 at a convergent point of multiple oncogenic pathways for cancer therapy. Nat. Commun. 5:5476 doi: 10.1038/ncomms6476 (2014).